Adaptive rheology and ordering of cell cytoskeleton govern matrix rigidity sensing Matrix rigidity sensing regulates a large variety of cellular processes and has important implications for tissue development and disease. However, how cells probe matrix rigidity, and hence respond to it, remains unclear. Here, we show that rigidity sensing and adaptation emerge naturally from actin cytoskeleton remodelling. Our in vitro experiments and theoretical modelling demonstrate a biphasic rheology of the actin cytoskeleton, which transitions from fluid on soft substrates to solid on stiffer ones. Furthermore, we find that increasing substrate stiffness correlates with the emergence of an orientational order in actin stress fibres, which exhibit an isotropic to nematic transition that we characterize quantitatively in the framework of active matter theory. These findings imply mechanisms mediated by a large-scale reinforcement of actin structures under stress, which could be the mechanical drivers of substrate stiffness-dependent cell shape changes and cell polarity. Living cells probe the rigidity of their environment as they anchor and pull on their surrounding matrix. Their ability to sense extracellular matrix rigidity is crucial for many cellular processes including cell migration [1] , differentiation [2] , [3] and proliferation [4] . It has also been implicated in tissue development [5] , [6] and disease [7] , [8] , but a clear understanding of its underlying mechanisms is still lacking [9] . Several cellular structures, acting at different length scales, have been proposed as matrix rigidity sensors. They include integrin-mediated focal adhesions (FAs) [10] , [11] , ion channels [12] and actin cytoskeleton [13] , [14] , [15] . The study of integrin-mediated FAs, which are local mechanosensors, has been largely favoured to explain cell mechanosensing through the modulation of their binding activity under force [16] , [17] , [18] . Consequently, the idea of large-scale mechanosensing mechanisms driven by actin cytoskeleton reorganization was relegated to the backseat for a while. However, it has recently been revisited by experimental and theoretical studies [13] , [19] , [20] , [21] , suggesting that contractile actomyosin-based units can themselves act as rigidity sensors. Along the same line, the anchoring of a cell to the extracellular matrix involves cell shape changes that produce mechanical stresses not only in the matrix but also in the cell itself [22] , [23] , [24] . Recent evidence indicates that the stiffness of the external environment induces a remodelling of the actin cytoskeleton [20] , [25] , [26] , [27] , along with an adaptation of the internal elasticity of the cell [28] . However, the mechanical coupling between matrix rigidity and cellular mechanical properties by which cells could detect rigidity and modulate their behaviour remains unknown. Here we show experimentally, and argue theoretically, that substrate stiffness dictates the behaviour of actin cytoskeleton by tuning its rheological properties from fluid like to solid like as stiffness increases. Actin filament ordering increases with substrate stiffness To investigate the influence of substrate stiffness, and to measure cellular traction forces, we used micro-fabricated pillar substrates whose stiffness can be tuned by changing the height of the micropillars (inset; Fig. 1a ). We developed a novel experimental setup to enable use of high numerical aperture (NA) objectives with micropillar substrates for high-quality live-cell imaging ( Fig. 1 ; Methods). To observe changes in cell shape, FA distribution, and actin reorganization with varying substrate stiffness, we stained the actin cytoskeleton of YFP-Paxillin expressing rat embryonic fibroblast (REF-52) cells on substrates with stiffnesses of 9, 43, 64 and 85 nN μm −1 ( Fig. 2a–d ). On the soft substrate (9 nN μm −1 ), cells did not form stress fibre-like structures, and a large proportion of them presented a non-polarized circular shape with an orthoradial pattern of actin filaments around the nucleus ( Fig. 2a ). Moreover, most of the FAs in these cells were localized at the periphery ( Fig. 2i ), and were smaller (<1 μm 2 on average) compared with those on stiffer substrates ( Fig. 2j ). This observation, along with higher unbinding rate of integrins in FAs under low forces [17] , indicates low substrate friction on soft substrates. In contrast, we observed marked changes in cell shapes from a circular to a well-spread, polarized morphology when comparing the softest with the stiffest substrate (85 nN μm −1 ). Both the morphology of the cells and their cytoskeletal organization were significantly different on the substrates of 9, 43, 64 and 85 nN μm −1 . Cells became more elongated with increasing substrate stiffness ( Supplementary Fig. 1 ), and on the stiffest substrate we observed well-developed stress fibres, preferentially aligned in the same direction ( Fig. 2d ), showing a large-scale order as previously observed [20] , [26] . Although such large-scale order over the entire cell area in stress fibre organization was not observed at intermediate stiffnesses (43 and 64 nN μm −1 ), our analysis revealed the formation of microdomains of locally ordered actin stress fibres ( Fig. 2b,c ), whose size increased with substrate stiffness ( Fig. 2k ). We processed the images of cells stained with actin to measure the local angles of actin filaments (see Methods), which are represented as coloured orientation plots ( Fig. 2e–h ). The uniformly coloured regions clearly indicate the presence of actin microdomains ( Fig. 2f,g ). As the substrate stiffness increases, actin stress fibres appeared to cluster into larger and fewer locally ordered microdomains, resulting in a large-scale order for the stiffest substrates. To confirm that the obtained results were not specific to the discrete micropillar substrates, we carried out similar experiments on soft and rigid continuous substrates [29] of equivalent rigidities [30] (see Methods). Actin distribution on these continuous substrates confirmed our observations of orthoradial organization on soft substrates, and actin filament microdomains on stiff substrates ( Supplementary Fig. 2 ). As such, the emergence of cellular scale order in stress fibre organization, with increasing matrix rigidity, has common features with the isotropic-nematic transition observed at the molecular scale in nematic liquid crystals and nematic gels [31] , [32] , [33] . 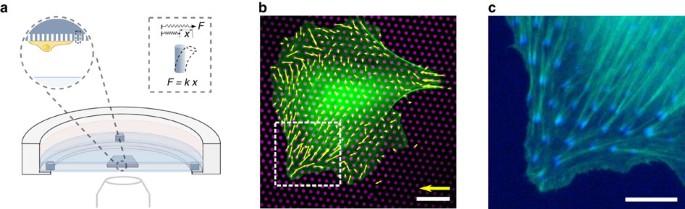Figure 1: (a) Schematic showing cross-section of the experimental setup for imaging cells in an upside-down configuration. The micropillar substrate can be seen between two coverslips. The inset shows a single micropillar on the substrate. Each micropillar behaves as a linear elastic spring. (b) Typical live-cell epi-fluorescent image of a rat embryonic fibroblast (REF-52) cell obtained using the setup. Cells expressYFP-PaxillinandRFP-Ftractin, which label focal adhesions and actin filaments (green), respectively. Underlying micropillar substrate (43 nN μm−1) is coated with fluorescent fibronectin (magenta) and corresponding traction force vectors are shown (yellow). Scale bars, 50 nN and 20 μm, respectively. (c) Image showing actin (green) and paxillin (blue) for the inset inb. Scale bar, 10 μm. Figure 1: ( a ) Schematic showing cross-section of the experimental setup for imaging cells in an upside-down configuration. The micropillar substrate can be seen between two coverslips. The inset shows a single micropillar on the substrate. Each micropillar behaves as a linear elastic spring. ( b ) Typical live-cell epi-fluorescent image of a rat embryonic fibroblast (REF-52) cell obtained using the setup. Cells express YFP-Paxillin and RFP-Ftractin , which label focal adhesions and actin filaments (green), respectively. Underlying micropillar substrate (43 nN μm −1 ) is coated with fluorescent fibronectin (magenta) and corresponding traction force vectors are shown (yellow). Scale bars, 50 nN and 20 μm, respectively. ( c ) Image showing actin (green) and paxillin (blue) for the inset in b . Scale bar, 10 μm. 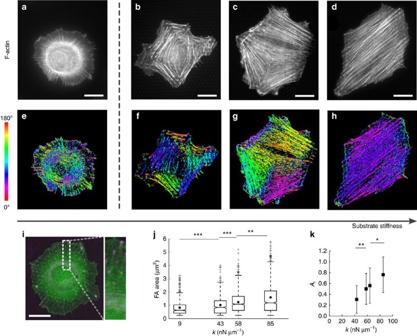Figure 2: Actin cytoskeleton and focal adhesion organization depends on substrate stiffness. (a–d) REF-52 cells stained for actin filaments (F-actin) on soft (9 nN μm−1—(a)) and stiff (43—(b), 64—(c) and 85nN μm−1—(d)) micropillar substrates. (e–h) Corresponding orientation plots for actin staining, where the different colours indicate different orientations of actin filaments as per the given colourmap. Actin stress fibre microdomains can be identified by the uniformly coloured zones in the orientation plots. (i) Live-cell image of REF-52 cell transfected withRFP-Ftractin(green) andYFP-Paxillin(magenta), on soft substrate (9 nN μm−1). (j) Focal adhesion (FA) area as function of substrate stiffness,k. Each boxplot corresponds to at least 500 FAs from five cells.• represents the mean areas. Box ends represent the first and third quartiles of the data, and whisker ends represent the last data within 1.5 interquartile range. (k) Area of actin microdomains relative to cell area,Ar, as a function of substrate stiffness,k. Each data point represents 25–30 cells and error bars represent s.e. of mean.Pvalues were calculated using Mann–WhitneyU-test. *P<0.05;**P<0.01;***P<0.0001. Scale bars, 20 μm. Full size image Figure 2: Actin cytoskeleton and focal adhesion organization depends on substrate stiffness. ( a – d ) REF-52 cells stained for actin filaments (F-actin) on soft (9 nN μm −1 —( a )) and stiff (43—( b ), 64—( c ) and 85nN μm −1 —( d )) micropillar substrates. ( e–h ) Corresponding orientation plots for actin staining, where the different colours indicate different orientations of actin filaments as per the given colourmap. Actin stress fibre microdomains can be identified by the uniformly coloured zones in the orientation plots. ( i ) Live-cell image of REF-52 cell transfected with RFP-Ftractin (green) and YFP-Paxillin (magenta), on soft substrate (9 nN μm −1 ). ( j ) Focal adhesion (FA) area as function of substrate stiffness, k . Each boxplot corresponds to at least 500 FAs from five cells.• represents the mean areas. Box ends represent the first and third quartiles of the data, and whisker ends represent the last data within 1.5 interquartile range. ( k ) Area of actin microdomains relative to cell area, A r , as a function of substrate stiffness, k . Each data point represents 25–30 cells and error bars represent s.e. of mean. P values were calculated using Mann–Whitney U -test. * P <0.05; ** P <0.01; *** P <0.0001. Scale bars, 20 μm. Full size image Actin rheology is regulated by substrate stiffness We further investigated actin cytoskeleton remodelling for soft and stiff substrates by live-cell imaging using our experimental setup ( Fig. 1 ). On the soft substrate, we observed a radial flow of actin filaments for the circular cells ( Supplementary Movie 1 ). The cell morphology and radial flow were stable during our observation time (at least 2 h). In contrast, on the stiff substrate (85 nN μm −1 ), we observed prominent stress fibres ( Fig. 3b ) that were stabilized shortly after formation. To quantify the spatio-temporal evolution of actin within the cells, we plotted kymographs of actin intensity. These kymographs clearly show an actin flow directed from the cell edge towards the cell centre on the soft substrare, and almost no motion of actin relative to the substrate on stiff substrates ( Fig. 3a–c ). Thus, we conclude that stable actin structures were promoted on stiff substrates over timescales similar to the ones used for the analysis on soft substrates. Presence of actin flow on soft substrates, and its absence on stiff substrates over similar timescales, strongly suggest that the cytoskeleton can be described as fluid-like material on soft substrates, and solid-like material on stiffer substrates. 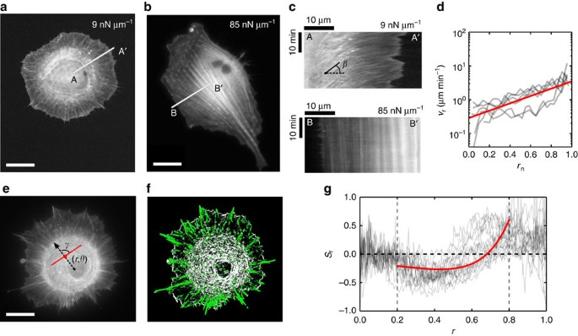Figure 3: Viscous behaviour of cells on soft substrates. (a,b) Live-cell image of REF-52 cell transfected withRFP-Ftractin, on soft (9 nN μm−1) and stiff (85 nN μm−1) substrates, respectively.RFP-Ftractinlabels actin filaments. (c) Kymographs along lines AA′ and BB′ inaandb, respectively. The kymographs show presence of flow of actin on soft substrate. The cells were imaged every 10 s for 25 min. (d) Radial velocity of actin filaments,vr=1/tanβas a function ofrn, whereβis the angle as indicated inc. Experimental data (grey) was obtained from six cells. Theoretical fit (red) forvrwas obtained fromSupplementary Equation 6usingvp=3.5 μm min−1andR/a=2.5. (e) REF-52 cell immunostained for actin filaments onk=9 nN μm−1;γis the angle between actin filament at (r,θ) and the radial vector. (f) Corresponding colour-coded image obtained after image analysis; green indicates radial arrangement (γ<45°), and white indicates orthoradial arrangement (γ>45°). (g) Actin order parameter in polar coordinates,Sr(r)=〈cos(2γ)〉. Experimental data (gray) was obtained from 17 cells. Theoretical fit (red) forSrwas obtained fromSupplementary Equation 13usingR=30 μm,R1=0.8R,R/a=2.5,vp=3.5 μm min−1,α=6.5 andβ1=0.7. Vertical dashed lines atr=0.2 andr=0.8 correspond torn=0 andr=R1, respectively. Scale bars, 20 μm. Figure 3: Viscous behaviour of cells on soft substrates. ( a , b ) Live-cell image of REF-52 cell transfected with RFP-Ftractin , on soft (9 nN μm −1 ) and stiff (85 nN μm −1 ) substrates, respectively. RFP-Ftractin labels actin filaments. ( c ) Kymographs along lines AA′ and BB′ in a and b , respectively. The kymographs show presence of flow of actin on soft substrate. The cells were imaged every 10 s for 25 min. ( d ) Radial velocity of actin filaments, v r =1/tan β as a function of r n , where β is the angle as indicated in c . Experimental data (grey) was obtained from six cells. Theoretical fit (red) for v r was obtained from Supplementary Equation 6 using v p =3.5 μm min −1 and R / a =2.5. ( e ) REF-52 cell immunostained for actin filaments on k =9 nN μm −1 ; γ is the angle between actin filament at ( r , θ ) and the radial vector. ( f ) Corresponding colour-coded image obtained after image analysis; green indicates radial arrangement ( γ <45°), and white indicates orthoradial arrangement ( γ >45°). ( g ) Actin order parameter in polar coordinates, S r ( r )=〈cos(2 γ )〉. Experimental data (gray) was obtained from 17 cells. Theoretical fit (red) for S r was obtained from Supplementary Equation 13 using R =30 μm, R 1 =0.8 R , R / a =2.5, v p =3.5 μm min −1 , α =6.5 and β 1 =0.7. Vertical dashed lines at r =0.2 and r =0.8 correspond to r n =0 and r = R 1 , respectively. Scale bars, 20 μm. Full size image For the soft substrates, we used the obtained kymographs to compute the average radial velocity of actin flows as a function of the distance from the inner edge of orthoradial fibres. This revealed an exponentially decaying flow starting with a fast retrograde flow at the cell leading edge (≈3.5 μm min −1 ) and terminating with slowly moving circular contractile actin cables that converge and stop near the cell nucleus ( Fig. 3d ). These results show that, on soft substrates, the actin structures nucleated at the cell periphery are advected across the cell, and are disassembled within a lifetime of the order of minutes, significantly shorter than typical observation timescales (>30 min). On soft substrates, the observed circular cell shape ( Fig. 3a ) is, thus, correlated with a prominent centripetal actin-remodelling flow towards the cell centre, together with small and isotropic adhesion complexes (<1 μm 2 on average) mostly distributed at the cell edge ( Fig. 2i,j ). This unanticipated response could, thus, be interpreted as a fluid-like behaviour of the cytoskeleton driven by a dissipative contractile actin flow. The conventional understanding of cell cytoskeletal behaviour as a function of substrate stiffness has been mainly based on the idea that cell elasticity could match the one of the underlying substrate [28] , [34] . The results presented here show this viewpoint to be incomplete. It appears that not only the elastic but also the viscous responses can be tuned by substrate stiffness. To test this interpretation further, we directly measured the fluidity of these cells on both the soft and stiff substrates. We used atomic force microscope (AFM) to perform creep tests on cells adhered to the soft (9 nN μm −1 ) and stiff (85 nN μm −1 ) micropillar substrates (see Methods). We found that the cells are more fluid on the soft substrates compared with the stiff substrates ( Supplementary Fig. 3 ). Altogether, our findings show that increasing substrate stiffness can result in switching of the dynamical mechanical properties of the actin cytokeleton from fluid like to solid like. Isotropic to nematic transition of the actin cytoskeleton Our results put forward a physical picture in which substrate stiffness triggers the rheological responses of the cell cytoskeleton. To evaluate whether these cellular responses can be captured in the framework of viscoelastic active materials [32] , we developed a two-dimensional theoretical model based on active gel theory [35] , [36] , which has proved to be a powerful tool to analyse cytoskeleton dynamics and model cell mechanics [37] . We described the actin cytoskeleton starting from a linear Maxwell model of viscoelasticity, considered here in two dimension, which relates the passive stress in the gel (that is, in the absence of myosin motors) to the strain rate tensor (see Supplementary Note 1 ). This model involves a single relaxation time τ , which is characterized by the typical lifetime of actin structures in the cytoskeleton. In this model, at timescales << τ , actin structures are conserved and the cytoskeleton behaves as a linear elastomer; at timescales >> τ , the cytoskeleton behaves as a Newtonian fluid. We argue below that this description, where τ is taken to crucially depend on substrate stiffness, explains our observations well. Soft substrates . On soft substrates, our observations showed that the lifetime of actin structures is smaller than the observation timescale ( Fig. 3c ). Therefore, we assumed τ to be small on soft substrates and considered the limit of a viscous nematic active gel. The orientational ordering of actin filaments is measured by the nematic order parameter Q ij =〈 n i n j − δ ij /2〉, where the average is taken over the local orientation of actin filaments, characterized by a unit vector n i (we will also make use of the scalar order parameter ). Following active gel theory [38] , the contractile effect of myosin motors is described by an active contribution to the stress tensor , where ζ and ζ ′ are phenomenological coupling constants, such that the total stress tensor is finally given by . Following classical arguments of hydrodynamics of liquid crystals [39] , the dynamics of nematic order parameter are coupled with the strain rate tensor, which in the regime of fast relaxation takes the simple form [38] : where α is a positive phenomenological coupling constant and v r denotes the radial component of the actin flow velocity. Making use of force balance, an explicit form of velocity profile can be derived (see Supplementary Note 1 ), which takes a simple exponential form: for r ∼ R , where R denotes the cell radius and v p is the actin polymerization velocity at cell edge. Notably, this functional form of the velocity is characterized after rescaling by a single parameter, the friction length (where ξ is the friction and η the gel viscosity), which was used to fit the data. A good agreement with the experimental data was found ( Fig. 3d ), and yielded that a is of the order of the cell size. This shows that friction is effectively low on soft substrate, which is consistent with our observation that strong FAs can form only on stiff substrates ( Fig. 2j ), and earlier observations that they have higher unbinding rates at low forces [17] . In addition, we found that flow alignment effects and boundary polymerization are sufficient to explain the observed orthoradial actin organization ( Supplementary Equation 13 ; Fig. 3e–g ), which in the absence of active drive (contractility or actin polymerization) would be isotropic in this regime. Although the flow alignment effects here are identical to those of passive nematic liquid crystals, activity is crucial to generate the actin flow [40] . Here, we have focused on actin polymerization at the cell periphery, which proved to be sufficient to fit the data but gradients of myosin-induced contractility ( Supplementary Fig. 4 ) are also expected to contribute to the actin flow. They could be taken into account in the model by making ζ and ζ ′ space dependent. Finally, the good agreement of both flow and order parameter profiles with experimental data indicates that the actin cytoskeleton can be described as a viscous nematic gel on soft substrates. Stiff substrates . On the stiff substrates, the lifetime of actin structures was greater than observation times ( Fig. 3c ). Therefore, we considered the large τ limit of the model on stiff substrates, according to which the cytoskeleton behaves as an elastic nematic gel. To investigate the emergence of order at the cellular scale, the nematic order parameter tensor Q was defined, following [26] , as averaged over the whole cell in this regime. For an equilibrium elastic nematic gel, the strain tensor, , which quantifies the gel deformation, and the nematic tensor, Q , are generically coupled through a Landau free energy functional [31] that can be written to lowest order in , Q as: where γ , ρ c , ω and μ are coupling constants and denotes the usual quadratic elastic free energy. We note that terms in gradients of Q , as well as boundary terms, do not appear in the present mean field discussion in which Q is averaged over the cell. In addition, topological defects and domain walls, which could be responsible for the absence of large-scale order on soft substrates, are only effectively taken into account in our approach. Here ρ is linear in and can be interpreted as the effective gel density: , where ρ 0 and χ are phenomenological coupling constants. Note that formally, the S 2 term in Equation 1, which favours stress fibres alignment for ρ > ρ c , is comparable to the interaction term between stress fibres introduced in ref. 27 . However, it had a different physical origin there since it originated from elastic interactions in the cytoskeleton. For the sake of simplicity, we assumed that the order parameter S is obtained by minimizing , as in equilibrium, and that the cell interacts with the substrate only through the FAs located at the cell periphery ( Fig. 4a ). The displacement field of the cytoskeleton at the cell periphery is, therefore, related to the local deformation of pillars. 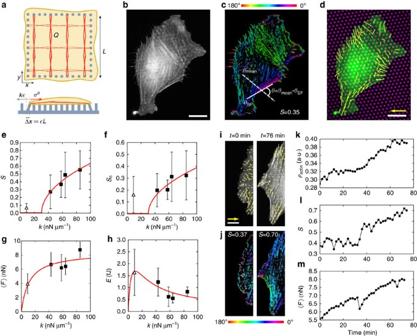Figure 4: Elastic behaviour of cells on stiff substrates. (a) Schematic of the theoretical model. (b) Live-cell image of a REF-52 cell labelled for actin on substrate withk=43 nN μm−1. Scale bar, 20 μm. (c) Corresponding orientation map for actin;θis the difference between the angle of a single actin filament,θSF, and the mean angle of all filaments,θmean. (d) Corresponding force vectors (yellow) are shown for actin-labelled cell (green) on its underlying micropillar substrate (magenta). Scale bars, 50 nN and 20 μm, respectively. (e) Order parameter of actin cytoskeleton,S=〈cos(2θ)〉 as a function ofk. Each data point represents 25–30 cells. Theoretical fit forSwas obtained fromSupplementary Equation 23usingk*=30 nN μm−1. (f) Order parameter of force vectors,Sσ, as a function ofk. (g) Mean traction force, 〈F〉, applied by cells as a function ofk. Theoretical fit for 〈F〉 was obtained fromSupplementary Equation 24usingcρ0=8.41 and 2χζ=11.49. (h) Mean energy per pillarEas a function ofk. Theoretical fit forEwas obtained fromSupplementary Equation 26usingc1=67,c2=15 and 2χζ=11.49. Each data point inf,g,hrepresents 8–11 cells imaged for 2 h, every 2 min. The error bars denote the s.e. of mean. Δ represents data for the soft substrate (9 nN μm−1), and ▪ represents data for stiff substrates (43, 58, 64 and 85 nN μm−1). (i) Actin stress fibre microdomain overlaid with corresponding force vectors (yellow) for a cell onk=43 nN μm−1. Scale bars, 40 nN and 15 μm, respectively. (j) Corresponding orientation plots. (k–m) Corresponding actin density (mean actin intensity),ρ, actin order parameter,S, and mean traction force, 〈F〉, as a function of time. Neglecting the passive contribution to stress, force balance is given by: Figure 4: Elastic behaviour of cells on stiff substrates. ( a ) Schematic of the theoretical model. ( b ) Live-cell image of a REF-52 cell labelled for actin on substrate with k =43 nN μm −1 . Scale bar, 20 μm. ( c ) Corresponding orientation map for actin; θ is the difference between the angle of a single actin filament, θ SF , and the mean angle of all filaments, θ mean . ( d ) Corresponding force vectors (yellow) are shown for actin-labelled cell (green) on its underlying micropillar substrate (magenta). Scale bars, 50 nN and 20 μm, respectively. ( e ) Order parameter of actin cytoskeleton, S =〈cos(2 θ )〉 as a function of k . Each data point represents 25–30 cells. Theoretical fit for S was obtained from Supplementary Equation 23 using k *=30 nN μm −1 . ( f ) Order parameter of force vectors, S σ , as a function of k . ( g ) Mean traction force, 〈 F 〉, applied by cells as a function of k . Theoretical fit for 〈 F 〉 was obtained from Supplementary Equation 24 using cρ 0 =8.41 and 2 χζ =11.49. ( h ) Mean energy per pillar E as a function of k . Theoretical fit for E was obtained from Supplementary Equation 26 using c 1 =67, c 2 =15 and 2 χζ =11.49. Each data point in f , g , h represents 8–11 cells imaged for 2 h, every 2 min. The error bars denote the s.e. of mean. Δ represents data for the soft substrate (9 nN μm −1 ), and ▪ represents data for stiff substrates (43, 58, 64 and 85 nN μm −1 ). ( i ) Actin stress fibre microdomain overlaid with corresponding force vectors (yellow) for a cell on k =43 nN μm −1 . Scale bars, 40 nN and 15 μm, respectively. ( j ) Corresponding orientation plots. ( k – m ) Corresponding actin density (mean actin intensity), ρ , actin order parameter, S , and mean traction force, 〈 F 〉, as a function of time. Full size image where is the active stress, K is proportional to substrate stiffness, k , and is the cellular strain (see Supplementary Note 1 ). Note that here the cellular strain was defined as the strain of stress fibres that are directly connected to the substrate, which can be quantified by the deformation of the pillars where stress fibres end. Thus, according to equation (4), substrate stiffness couples cellular strain with active stress, and therefore to the order parameter, S , according to the equation , where the dependence on density is made explicit. In fact, we found experimentally that during the assembly of an actin microdomain, the mean total force that it exerts on the substrate, 〈 F 〉, is proportional over time to its mean actin density, ρ ( Fig. 4i–m ; Supplementary Fig. 5 ). This supports our interpretation of ρ , introduced as a phenomenological coupling term, as indeed being the density of actin stress fibres, and it confirms the dependence of the active stress on ρ . We found that the coupling between substrate stiffness and order induced by the gel activity is responsible for a substrate stiffness-dependent transition from isotropic to nematic order at the cellular scale, formally similar to lyotropic liquid crystals. The transition occurs at a critical stiffness k *, equivalent to a critical density ρ *: for k < k *, S =0 and the system is isotropic at the cellular scale, while for k > k *, the radial symmetry is spontaneously broken and S >0 (see Supplementary Note 1 ). This provides a simple stiffness-dependent ordering mechanism, which is in qualitative agreement with our observations. As in classical second-order phase transitions, this analysis predicts that close to the transition, one has , which agrees well with observations ( Fig. 4e ). The theoretically obtained transition stiffness k *=30 nN μm −1 (≈21 kPa [30] ) is similar to the in vivo environment of cells in tissues such as cartilages ( E ≈20 kPa) [41] . Thus, such isotropic-nematic transition could have implications for behaviour of these cells in vivo . We point out that finite size effects are very important at the cell scale, and some expected features of second-order phase transitions, such as power decay of correlation functions, cannot be directly tested here. However, we did find that the correlation length of the local order parameter increases with substrate stiffness ( Supplementary Fig. 6 , see Methods). Also, we stress that although the coupling between actin alignment, S , and strain, , as introduced in equation (1), is formally the same as in passive nemato-elastomers [31] , activity plays a central role here. It is taken into account in the active stress (which is coupled with substrate stiffness through force balance), and in the dependence of actin density, ρ , on strain, . Indeed, the transition to nematic order, as is observed experimentally, can be obtained only for χ >0, which is a hallmark of non-equilibrium processes: as opposed to passive materials at equilibrium, for which χ <0, here actin density increases for smaller compressive strain. This behaviour, which we report at the cell scale, is comparable to that of FAs, whose area increases on less deformable substrates [25] , [42] ( Fig. 2j ). Finally, the transition can be qualitatively described as follows. On a soft substrate, the active stress is sufficient to induce large strain; the actin density remains low, and as in lyotropic liquid crystals, the phase is isotropic. On stiff substrates, the strain is small and actin density is increased; if a critical value is reached, nematic order appears and the stress becomes anisotropic. Our results show that on stiff substrates actin cytoskeleton can be well described as an elastic nematic gel, which undergoes a transition from isotropic to nematic order at the cellular scale. In conclusion, our experimental and theoretical findings establish a quantitative picture of the mechanisms that drive cell response to substrate rigidity. We show that the process of substrate stiffness mechanosensing is governed by a much more versatile switch of the rheological properties of actin cytoskeleton than previously thought. Our study reveals that the actin cytoskeleton, as a rigidity sensor, behaves as a fluid-like material on soft substrates and as a solid-like material on stiffer ones, with the solid behaviour characterized by a transition from isotropic to nematic order at the cellular scale leading to higher order and higher tension on stiffer substrates ( Fig. 5 ). 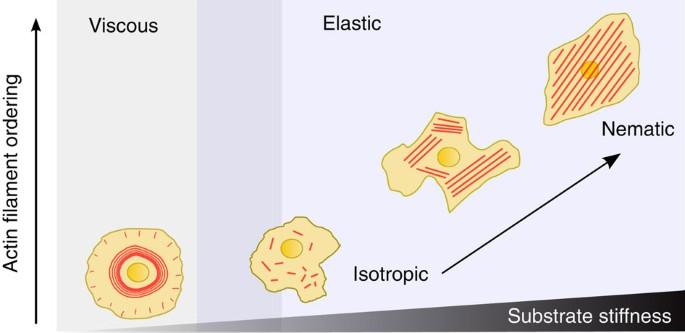Figure 5: Evolution of cell rheology and actin organization with substrate stiffness. As the substrate stiffness inceases, the large-scale order of actin filament alignment also increases. On soft substrates, actin cytoskeleton shows viscous behaviour, whereas on stiff substrates it shows elastic behaviour. On stiff substrates, as the stiffness increases, the cytoskeleton undergoes an isotropic to nematic phase transition. Figure 5: Evolution of cell rheology and actin organization with substrate stiffness. As the substrate stiffness inceases, the large-scale order of actin filament alignment also increases. On soft substrates, actin cytoskeleton shows viscous behaviour, whereas on stiff substrates it shows elastic behaviour. On stiff substrates, as the stiffness increases, the cytoskeleton undergoes an isotropic to nematic phase transition. Full size image The viscoelastic transition could be related to the dynamics of FAs on soft and stiff substrates. On soft substrates FAs are short-lived [17] , [18] , which implies a low-friction with the substrate. Since FAs serve as mechanical links between actin cytoskeleton and the underlying substrate, this low friction favours actin flows in response to contractile stress. This, in turn, contributes to destabilizing FAs, and more generally cross-linked actin structures, leading to a small viscoelastic timescale τ . In contrast, solid-like behaviour on stiffer substrates implies longer relaxation times, sufficient to promote FA assembly and more generally to stabilize cross-linked actin structures, consistent with a longer τ . This suggests that actin remodelling through force generation and FA assembly could involve a feedback loop that drives rigidity mechanosensing. In contrast to passive nemato-elastomers, our findings show that the actin density is increased for smaller strain (that is, on stiffer substrate), which is the signature of active processes. Such stabilization of actin structures under stress, already described in the context of FAs [25] , [43] , [44] , may be mediated at the scale of the cytoskeleton by the recruitment of both actin and its cross-linkers when order is increased. Furthermore, at the cellular scale on soft substrates, low-friction forces, and radial flow of actin favour circular cellular shapes, and consequently, non-motile behaviour of cells. In contrast, as stiffness increases, the assembly of stable stress fibres and their large-scale polarization induce cell shape changes and could promote polarity axis formation. Consequently, such behaviour could explain the ability of cells to move towards stiffer environments [1] . The low-friction regime observed on soft substrates prevents the formation of actin stress fibres, and as such, cell’s ability to generate high traction forces. This type of actin organization on soft substrates has been observed in neuronal growth cones [45] , and in cells cultured on cadherin-coated substrates [46] . Interestingly, neurons evolve in soft environments [5] , and cells exert less forces on cadherin-coated compared with fibronectin-coated substrates [47] . Thus, our findings on rigidity sensing may be extended to other mechanosensing processes. In conclusion, the cytoskeleton adaptation to substrate stiffness reported here is qualitatively distinct from any previous observation, and reflects a large-scale mechanosensing remodelling. As such, it suggests that substrate stiffness could modify cytoskeleton properties to fine-tune cell polarity and migration during development, and pathological processes such as metastasis [8] . Preparation and calibration of micropillar substrates The micropillar substrates were prepared from polydimethylsiloxane (PDMS, Sylgard 184, Dow Corning) elastomer using silicon wafers. The micropillars were 2 μm in diameter, with heights 3–9 μm, resulting in substrate stiffnesses of 9–85 nN μ m −1 . The micropillar tops were selectively coated with fluorescent dye-conjugated fibronectin (ATTO647N, Sigma-Aldrich) using microcontact printing technique—flat PDMS stamps were inked with 50 μg ml −1 fibronectin and 5 μg ml −1 dye-conjugated fibronectin; the stamps were then dried and placed on ultraviolet/ozone-treated micropillar substrates for 5 min. The softer substrates were immersed in 100% EtOH, rinsed with and reimmersed in PBS before stamping to prevent micropillar collapse. The substrates were then immersed in 0.2% Pluronics-F127 solution for 1 h to prevent cell adhesion to the micropillar sides, and then rinsed with PBS. PBS was then exchanged with cell culture medium to culture the cells. PDMS (1:10 cross-linker to base polymer ratio) was consistently cured at 80 °C for 2 h to obtain a Young’s Modulus, E =2 MPa. The dimensions of the micropillars were obtained from scanning electron microscope images. Finite element method was used to calculate the stiffness of the micropillars, using commercially available software package ABAQUS (SIMULIA, Dassault Systèmes). A micropillar was modelled as a neo-Hookean hyperelastic cylinder with E =2 MPa and was discretized into hexahedral mesh elements. The micropillar was placed on a base of the same material to account for substrate warping effects. Different forces were applied at the micropillar top, and corresponding top displacements were obtained. Micropillar stiffness was then obtained from slope of the resulting force-displacement curve. Preparation of polyacrylamide gel substrates Polyacrylamide (PAA) solution was prepared in HEPES with various ratios of 40% acrylamide and 2% bisacrylamide for desired stiffness [48] . N -hydroxisuccinimidil was added for protein binding, and amonium persulfate and N , N , N , N -tetramethylenediamine were added to facilitate gel polymerization. Twenty microlitre of this PAA solution was added onto 22-mm coverslip (silanized with Bindsilane, acetic acid and ethanol (1:1:7)), and flattend with a fibronectin-stamped coverslip (similar to the method for micropillar substrates). This ensured adsorption of fibronectin on the PAA gel. The gel was allowed to polymerize for 30 min before removing the stamped coverslip and incubating the substrate in PBS. PBS was exchanged with cell culture medium for culturing cells. Cell culture and staining Rat embryonic fibroblast cells (REF-52), stably expressing YFP-Paxillin (gift from A. Bershadsky, Weizmann Institute, Israel), were maintained at 37 °C in a humidified atmosphere of 5% CO 2 and 95% air in Dulbecco’s modified Eagle medium (DMEM) containing 10% fetal bovine serum, 100 U ml −1 penicillin, 100 μg ml −1 streptomycin and 100 μg ml −1 glutamine. For live-cell observations of actin cytoskeleton, the cells were transfected with RFP-Ftractin [49] using electroporation (Nucleofactor, Lonza) to label actin filaments. Cells on micropillar substrates were fixed 3–4 h after seeding. They were fixed for 10 min at room temperature using 4% formaldehyde (PFA) in PBS, permeabilized using 0.1% Triton-X for 5 min, blocked for 1 h with 1% BSA in PBS and rinsed with PBS. Filamentous actin was stained with 10 μg ml −1 Phalloidin-TRITC (Sigma-Aldrich) for 20 min. Fluorescence microscopy Fluorescent live-cell and fixed-cell images were obtained using an Olympus IX81 inverted epifluorescence microscope equipped with an Olympus UPLSAPO 60 × W/1.2 NA objective, and a box and temperature and CO 2 controller (Life Imaging Sciences). Live-cell imaging was performed 3–4 h after seeding the cells on the micropillar substrates. An imaging setup was developed to enable use of the high NA objective with micropillar substrates for high-quality live-cell imaging of actin cytoskeleton. Briefly, the micropillar substrate with live cells was mounted on a glass coverslip, which was then inverted over another coverslip with spacers of thin (≈300 μm) silicone membranes (Specialty Manufacturing Inc., USA), preventing the cells from getting squeezed. The coverslips were mounted in a holder (Bioptechs Inc., USA) for imaging. Live-cell images were taken every 10 s or 2 min for 30 min or 2 h, respectively. Leibovitz’s L-15 cell culture media (Life Technologies) supplemented with 10% fetal bovine serum was used to minimize background. AFM experiments and analysis Fluidity of cells was calculated from creep indentation measurements on live cells adhered to soft (9 nN μm −1 ) and stiff (85 nN μm −1 ) micropillar substrates. To indent the cells, we used a NanoWizard AFM (JPK Instruments, Germany), with a silicon nitride cantilever (nominal spring constant of 30 nN μm −1 ), and a spherical silica bead of diameter 4.5 μm attached to its tip. A step load of 1 nN was maintained for at least eight points on each cell for 10 s, and the change in the z-sensor signal was measured. The obtained creep curves were fitted with standard linear solid model to obtain the fluidity (1/ η 1 ) of the cells, using the equation: where, is the strain in the cell and σ 0 is the constant loading stress. Ten cells were probed for each of the two stiffnesses. Micropillar deflection calculation Live-cell images were used to calculate the deflection maps for the micropillar substrates. The fluorescent images of micropillar tops were analysed using a custom-built ImageJ plugin. Briefly, the micropillar centroids were detected with subpixel resolution using a circular Gaussian filter, and then tracked for all the frames of the obtained time-lapse movies. The deflection of the mircropillars was calculated by estimating the rest positions of the micropillars and finding their difference with the corresponding micropillar centroid position. A grid of micropillar positions corresponding to known dimensions of the undeflected substrate was fitted to the images for this purpose. The obtained data were further analysed in a custom python program to calculate traction forces. Actin order parameter calculation The images of fluorescent actin cytoskeleton were analysed using a custom-built MATLAB program. Briefly, the local orientation of actin at each pixel in the image was calculated by obtaining the structure tensor of the image. Then, the order parameter, S =〈cos(2 θ )〉, where θ is the difference between local fibre orientation and average fibre orientation for a given cell, was calculated. Actin order parameter in polar coordinates, S r ( r ) was calculated by measuring the angle γ between the actin filament at each point ( r , θ ) and radial vector from cell centre ( Fig. 3e ). The local angles of filaments were obtained from structure tensor of the image. S r ( r ) was then calculated using S r =〈cos(2 γ )〉, where the average is taken over all θ for an r . Measurement of actin filament orientation autocorrelation Images of fluorescently labelled actin filaments were analysed using a custom-built ImageJ plugin. Local orientation of actin filaments at each pixel in the image was calculated by obtaining the structure tensor of the image. The obtained angles were averaged in a region of 25 × 25 pixels (1 px=0.111 μm). Graphical representation of these angles is presented in Supplementary Fig. 6 as yellow lines. Spatial autocorrelation of these averaged angles was calculated as A ( r )=〈cos2( θ i − θ j ( r ))〉, where 0< r <40 μm. Forty micrometre is the approximate average cell radius. Measurement of FA area First, images of cells with fluorescently labelled paxillin were smoothed using a Gaussian filter. Then, background was removed using ‘rolling ball’ backgroud subtraction algorithm in ImageJ, with a ball diameter of 50 pixels (1 px=0.111 μm). The image was then thresolded, and resulting particles were analysed to obtain their area. Any FAs with area <0.15 μm 2 were removed from the data. Measurement of actin intensity in cells Average intensity of cells was calculated using the area covered by cells as a mask, and subtracting average pixel intensity outside this mask from the pixels inside the mask. Pixel intensities were thresholded in ImageJ to obtain the mask. How to cite this article : Gupta, M. et al . Adaptive rheology and ordering of cell cytoskeleton govern matrix rigidity sensing. Nat. Commun. 6:7525 doi: 10.1038/ncomms8525 (2015).